syn-Selective alkylarylation of terminal alkynes via the combination of photoredox and nickel catalysis Substituted alkenes are pivotal structural motifs found in pharmaceuticals and agrochemicals. Although numerous methods have been developed to construct substituted alkenes, a generally efficient, mild, catalytic platform for the conversion of alkynes to this highly functionalized scaffold via successive C–C bond forming steps remains in high demand. Here we describe an intermolecular, regio- and syn -stereoselective alkylarylation of terminal alkynes with tertiary alkyl oxalates via photoredox-Ni dual catalysis. This catalytic protocol, synergistically combining Ir/Ni-catalyzed alkyne difunctionalization with photoinduced alkene isomerization, affords trisubstituted alkenes with excellent efficiency and syn -stereoselectivity. The mild conditions tolerate many functional groups, allowing for a broad scope with respect to terminal alkynes, aryl bromides, and alkyl oxalates. Substituted alkenes are pivotal structural motifs found in pharmaceuticals, agrochemicals, and biologically active natural products [1] , [2] , [3] , as well as versatile synthetic building blocks in organic synthesis [4] , [5] . Consequently, the development of general protocols for the regio- and stereoselective synthesis of alkenes, particularly employing readily available and abundant precursors, is a long-standing goal of chemical synthesis [6] , [7] . Transition metal-catalyzed direct functionalization of alkynes is a powerful method to access substituted alkenes with stereoselectivity control [8] , [9] , [10] , [11] , [12] , [13] , [14] , [15] , [16] , [17] , [18] , [19] , [20] , [21] . Generally, two distinct strategies have been utilized: one is a catalytic generation of syn -substituted alkenyl metal species, via migratory insertion controlled by the stereoelectronic effect, followed by protonation or coupling to deliver trisubstituted alkenes with syn -stereoselectivity [8] , [9] , [10] , [11] , [12] , [13] , [14] , [15] , [16] , [17] , [18] , [19] , [20] , [21] , [22] , [23] , [24] , [25] , [26] , [27] , [28] ; the other is transition metal-catalyzed radical addition/coupling reaction of alkynes, typically favoring anti -addition which is dominated by steric factors of vinyl radicals in the coupling step (Fig. 1 a) [29] , [30] , [31] , [32] , [33] , [34] , [35] , [36] , [37] . Although numerous methods have been developed toward addressing the challenge of regio- and stereo-selectively forming trisubstituted alkenes, a generally efficient, mild, catalytic platform for the conversion of alkynes to this highly functionalized scaffold via successive C–C bond forming steps would be highly demanding and represent a valuable advance in synthetic methodology. Fig. 1 syn -Alkylarylation of terminal alkynes via the combination of photoredox and nickel catalysis. a Alkyne functionalizations via transition metal catalysis. b syn -Alkylarylation of alkynes via metallaphotoredox catalysis Full size image Over the last decade, visible light photocatalysis have emerged as a powerful platform in organic synthesis by activating organic molecules through either single-electron transfer or energy transfer [38] , [39] , [40] , [41] , [42] , [43] . Particularly, the ability of the photoredox catalyst to modulate the oxidation state of organometallic species has enabled the efficient construction of challenging C–C bonds [44] , [45] , [46] , [47] , [48] , [49] . Recently, this solar-energy-driven catalytic technology has been utilized to facilitate contra-thermodynamic E → Z isomerization of olefins through an energy-transfer manifold, enabling the facile synthesis of Z -olefins [50] , [51] , [52] , [53] , [54] , [55] , [56] . We recently questioned whether metallaphotoredox catalysis could serve as an alternative platform to access trisubstituted alkenes with high control over stereoselectivity [57] , [58] , [59] . Specifically, a catalytic protocol including three sequential events, (i) alkyl radical addition to the C≡C bond [29] , (ii) cross-coupling of the resulting alkenyl radical with nickel complex, and (iii) photochemical E → Z isomerization of olefins, would deliver the stereodefined trisubstituted alkenes. We envisioned that the unique metallaphotoredox manifold would enable the generation of alkyl radicals from readily available feedstocks [60] such as alcohols [61] , and more importantly could be leveraged to enrich the stereoselectivity of alkyne addition reactions. Herein, we demonstrate the first example of alkylarylation of terminal alkynes employing simple tertiary alcohol derivatives and aryl halides through the synergistic merger of photoredox and nickel catalysis [62] , [63] , furnishing a wide array of trisubstituted alkenes with syn -stereoselectivity under mild conditions (Fig. 1b ). This photoredox protocol provides complementary reactivity and stereoselectivity to a previous nickel system with alkyl halides as radical precursors, which affords the trisubstituted alkenes with anti -stereoselectivity at elevated temperature (80–120 °C) [34] . Design plan Inspired by Overman and MacMillan’s oxalate half-ester chemistry [64] , we chose tertiary alkyl oxalates as the alkyl precursors for our proposed metallaphotoredox alkyne chemistry. Tertiary oxalate salts are bench stable, and can be easily prepared from corresponding, abundant tertiary alcohols. As depicted in Fig. 2 , we envisioned that a single-electron oxidation of tertiary alkyl oxalate 3 ( E 1/2 = + 1.28 V vs SCE in CH 3 CN for tert -BuOCOCO 2 Cs) [64] by photoexcited Ir[dF(CF 3 )ppy] 2 (dtbbpy)(PF 6 ) 1 ( E 1/2 [Ir *III /Ir II = + 1.21 V vs SCE in CH 3 CN] [65] should generate alkyl radical 4 upon loss of two molecules of CO 2 as well as reduced Ir(II) species 5 . Alkyl radical 4 is expected to undergo regioselective addition to terminal alkyne 6 to produce linearized alkenyl radical 7 due to resonance stabilization effect [29] . An anti -addition of the high-energy alkenyl radial 7 and Ni(0) 8 is expected to deliver the ( E )-alkenyl-Ni(I) species 9 [66] . Subsequent oxidative addition of ( E )-alkenyl-Ni(I) 9 with aryl bromide 10 would afford ( E )-alkenyl-Ni(III) complex 11 [34] , [67] , which undergoes a facile reductive elimination to produce substituted alkene 12 with concomitant generation of Ni(I) complex 13 . Single-electron transfer between Ir(II) 5 { E 1/2 [Ir III /Ir II = −1.37 V vs SCE in CH 3 CN]} [65] and Ni(I) 13 ( E 1/2 [Ni II /Ni 0 = −1.2 V vs SCE in DMF] [68] would regenerate ground-state Ir(III) 1 and Ni(0) to close the two catalytic cycles. Given the polarity of 12 , at this juncture, we hypothesized that a E → Z isomerization of 12 would be possible through a photoinduced energy transfer manifold [50] , [51] , [52] , [53] , [54] , [55] , [56] , delivering the desired alkene 14 with syn -stereoselectivity. Alternatively, another catalytic pathway involving oxidative addition of Ni(0) with aryl bromide 10 [62] , [63] , [69] , followed by trapping of the nucleophilic vinyl radical 7 by aryl-Ni(II) 15 to furnish the key Ni(III) intermediate 11 , is also plausible. Fig. 2 Proposed mechanism. Two possible reaction pathways proposed on the basis of previous literature Full size image Optimization study We examined the feasibility of this proposed metallaphotoredox alkyne protocol by employing 4- tert -butylphenylacetylene 16 and 4-bromobenzaldehyde 17 as standard substrates. 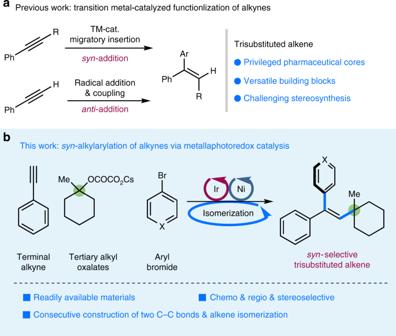Fig. 1 syn-Alkylarylation of terminal alkynes via the combination of photoredox and nickel catalysis.aAlkyne functionalizations via transition metal catalysis.bsyn-Alkylarylation of alkynes via metallaphotoredox catalysis As shown in Table 1 , upon irradiation by a 90 W blue LED of a solution of alkyne 16 , bromide 17 , and cesium oxalate 18 derived from 1-methyl-1-cyclohexanol in the presence of catalytic amounts of Ir[dF(CF 3 )ppy] 2 (dtbbpy)PF 6 1 , NiCl 2 •glyme, 4,4′-di- tert -butyl-2,2′-dipyridyl (dtbbpy) in DMSO, 81% yield of the desired trisubstituted alkene product 19 was obtained with excellent chemo-, regio-, and syn -selectivity ( Z / E = 96:4) (entry 1). The structurally similar photocatalyst Ir[dF(CF 3 )ppy] 2 (phen)PF 6 also promoted this transformation with moderate efficiency and excellent syn -selectivity (entry 2). Switching to other commonly employed photocatalysts, such as Ru(bpy) 3 (PF 6 ) 2 and 4CzlPN (2,4,5,6-tetra(9 H -carbazol-9-yl)isophthalonitrile), resulted in a dramatic decrease in efficiency (entries 3–4). The reaction proceeded with moderate to good efficiency in the presence of NiCl 2 (PPh 3 ) 2 or precatalyst NiCl 2 (Py) 4 (entries 5–6). The choice of solvent demonstrated a dramatic effect on the reaction efficiency, with DMSO proving to be optimal (entries 7–10). Interestingly, stereoselectivity of the alkene product appeared to be solvent independent (entries 7–10). 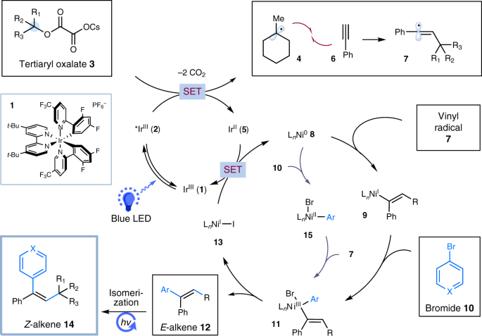Fig. 2 Proposed mechanism. Two possible reaction pathways proposed on the basis of previous literature Finally, control experiments demonstrated that light, photocatalyst, nickel catalyst, and ligand are all essential for the desired transformation to proceed (entries 11–14) (for additional control experiments, see Supplementary Tables 1 , 2 ). Table 1 Optimization of reaction conditions. a Full size table Substrate scope With optimal conditions in hand, we explored the generality of this metallaphotoredox protocol with respect to the alkyne fragment. As depicted in Fig. 3a , terminal arylalkynes bearing electron-neutral, -donating, and -withdrawing substituents proceeded smoothly under the optimal conditions, furnishing the corresponding trisubstituted alkenes with high to excellent yields and stereoselectivity (products 19 − 30 , 65−90% yields, > 95:5 syn -selectivity). Notably, halides (F, Cl, Br) on the aryl ring of alkynes remained untouched, offering valuable handles for further manipulations (product 24 − 29 , 65−90% yields, >91:9 syn -selectivity). Moreover, ortho substituents on the aryl ring had little effect to the reaction efficiency and selectivity (products 25 and 27 , 80% and 66% yield, >95:5 syn -selectivity, respectively). A slight erosion of yield and selectivity was observed when 3-ethynylthiophene was subjected to this multicomponent system (products 31 , 69% yield, 83:17 syn -selectivity). However, internal alkynes are not compatible in this reaction protocol, a result we attribute to increased steric hindrance. Fig. 3 Substrate scope. a Scope of alkynes. b Scope of cesium oxalates. c Scope of aryl halides. Reaction conditions: Ir- 1 (3 mol%), NiCl 2 •glyme (20 mol%), dtbbpy (20 mol%), alkyne (0.1 mmol), oxalate (1.5 equiv. ), bromide (2.0 equiv. ), DMSO [0.05 M], 90 W blue LED, 36 °C, 18 h. All cited yields are isolated yields. 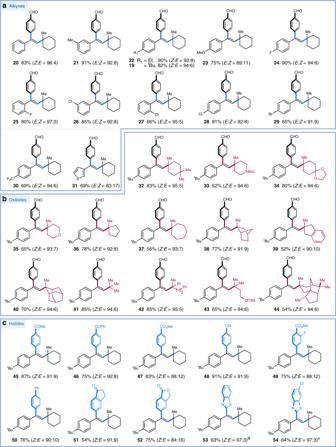Fig. 3 Substrate scope.aScope of alkynes.bScope of cesium oxalates.cScope of aryl halides. Reaction conditions: Ir-1(3 mol%), NiCl2•glyme (20 mol%), dtbbpy (20 mol%), alkyne (0.1 mmol), oxalate (1.5 equiv.), bromide (2.0 equiv.), DMSO [0.05 M], 90 W blue LED, 36 °C, 18 h. All cited yields are isolated yields. The ratios of the two isomers were determined by1H NMR analysis of the crude reaction mixtures.aHeteroaryl chloride was employed.dtbbpy= 4,4′-di-tert-butyl-2,2′-dipyridyl The ratios of the two isomers were determined by 1 H NMR analysis of the crude reaction mixtures. a Heteroaryl chloride was employed. dtbbpy = 4,4′-di- tert -butyl-2,2′-dipyridyl Full size image Next, we evaluated the scope of cesium tertiary alkyl oxalates in this protocol. As shown in Fig. 3b , a variety of tertiary cesium oxalates, readily prepared from the corresponding tertiary alcohols, can be successfully employed with high levels of efficiency and stereoselectivity. Cyclic oxalates, derived from cyclohexanols, cyclopentanols, and cycloheptanols, underwent the desired addition/coupling smoothly, yielding the ( Z )-selective trisubstituted alkenes with high efficiency (products 32 − 40 and 44 , 52−83% yields, Z/E up to 95:5). Heterocycles, in the form of tetrahydropyran and piperidine, were also viable substrates (products 33 and 35 , 52% and 65% yields, Z/E > 93:7). A number of polycyclic oxalates could be effectively employed without loss in yield and selectivity (products 34 , 38 − 40 , and 44 , 49−84% yields, Z / E up to 94:6). Moreover, this photoredox protocol could further be applied to acyclic tertiary oxalates, furnishing the desired alkenes in good yields and excellent stereoselectivity favoring syn -addition (products 41 − 43 , 65−85% yields, Z/E > 94:6). Notably, natural-product-derived substrates, such as cedrol oxalate, proved successful, indicating the potential utility of this mild protocol with complex molecules (products 44 , 54% yield, Z/E = 94:6). Finally, we turned our attention to the scope of aryl bromides that can participate in this catalytic protocol. As revealed in Fig. 3c , a variety of electron-deficient aryl bromides can be readily employed with high efficiency and moderate-to-high stereoselectivity (products 45 − 54 , 54−91% yields, Z/E up to 97:3). Many valuable functional groups, including ketones, esters, nitrile, and lactones were found to be well tolerated under the mild conditions (products 45 − 52 , 54−91% yields, Z/E up to 92:8). Gratifyingly, benzothiazole-derived heteroaromatic chlorides could be efficiently employed in this synergistic protocol without any loss in stereoselectivity, albeit with a slight decrease in yields (products 53 and 54 , 63% and 64% yields, Z/E = 97:3, respectively). At this stage in our studies on this metallaphotoredox protocol, the scope of aryl halides is currently limited to electron-poor and electron-neutral system, in which a conjugated substituent at the para position is crucial to achieve excellent syn -stereoselectivity control (see Supplementary Figs. 13 , 14 ). To highlight the synthetic utility of this metallaphotoredox difunctionalization manifold, a gram-scale reaction of alkyne 16 was performed. The reaction proceeded smoothly, affording the desired alkylarylation product 19 in 65% yield with excellent stereoselectivity ( Z/E > 98:2) (Fig. 4 ). Fig. 4 Reaction on large scale. Reaction condition: Ir- 1 (3 mol%), NiCl 2 •glyme (20 mol%), dtbbpy (20 mol%), alkyne (4 mmol), oxalate (1.5 equiv. ), bromide (2.0 equiv. ), DMSO [0.05 M], 90 W blue LED, 36 °C, 18 h. Isolated yield. The ratio of the two isomers were determined by 1 H NMR analysis of the crude reaction mixture. dtbbpy = 4,4′-di- tert -butyl-2,2′-dipyridyl Full size image Mechanistic studies To probe the reaction pathway of this metallaphotoredox three-component coupling protocol, we conducted a series of preliminary mechanistic experiments. Time course studies showed that yields steadily increased overtime, while high stereoselectivity was observed at the early stage, suggesting that stereoselectivity of this transformation might be catalyst-independent (Fig. 5a ). To probe the stereo-enrichment process, ( E )-alkene 41 was prepared and subjected to the photoinduced system (Fig. 5c ). In the presence or absence of photocatalyst 1 , ( E )- 41 underwent the isomerization to yield ( Z )- 41 with excellent efficiency, indicating that photocatalyst does not actually engage in the isomerization event (Fig. 5c ). As expected, no isomerization of 41 was observed in the absence of visible light (Fig. 5c ). On the basis of these results, we expected that trisubstituted alkene itself might act as a photosensitizer for this photochemical isomerization. This hypothesis was further confirmed by UV–Vis absorption spectrometry of ( E )- 41 , which exhibited considerable overlap with the blue LED spectrum (Fig. 5b ). Particularly, the ( E )-isomer showed strong bathochromic shift relative to the ( Z )-isomer (Fig. 5b ). Predictably, deconjugation of the π-system in the ( Z )-isomer product secures high levels of stereocontrol in this contra-thermodynamic, photoinduced E → Z isomerization (see Supplementary Fig. 3 for density functional theory (DFT)-based conformational analysis). Furthermore, reaction of oxalate 18 with alkyne 16 in the absence of aryl bromide afforded the alkene product 55 in 23% yield (Fig. 5d ), providing supporting for the addition of alkyl radical to alkyne step shown in Fig. 2 . Nevertheless, only a trace amount of tert -alkyl-aryl coupling product was observed in the reaction of oxalate 18 with aryl bromide 17 (see Supplementary Fig. 10 ). These results suggest that, under these metallaphotoredox conditions, tertiary alkyl radical would be more prone to undergo radical addition to alkyne, as opposed to capture by nickel species, probably due to steric hindrance [70] . Finally, we have prepared Ni(II) oxidative addition complex [69] , [71] 56 to evaluate an alternative pathway involving radical capture by aryl-Ni(II) species 15 (Fig. 2 ). Irradiation with a 90 W blue LED of a solution of isolated aryl-Ni II -Br 56 , alkyne 16 , and oxalate 18 in the presence of stoichiometric amount of photocatalyst 1 led to no formation of the desired trisubstituted alkene product (Fig. 5e ). The major byproduct was biaryl, which could be formed via homo-coupling from disproportionation of Ni(II) complex 56 (see Supplementary Fig. 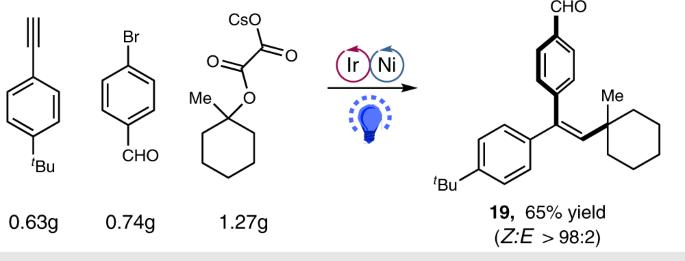Fig. 4 Reaction on large scale. Reaction condition: Ir-1(3 mol%), NiCl2•glyme (20 mol%), dtbbpy (20 mol%), alkyne (4 mmol), oxalate (1.5 equiv.), bromide (2.0 equiv.), DMSO [0.05 M], 90 W blue LED, 36 °C, 18 h. Isolated yield. The ratio of the two isomers were determined by1H NMR analysis of the crude reaction mixture. dtbbpy = 4,4′-di-tert-butyl-2,2′-dipyridyl 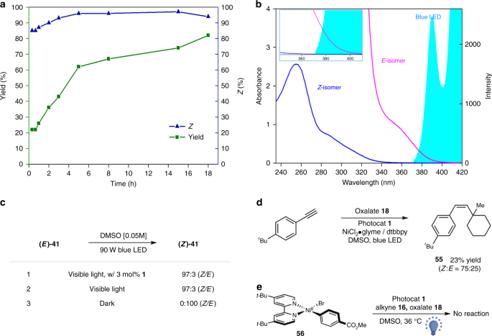Fig. 5 Mechanistic studies.aTime course studies;bUV–Vis absorption spectrometry;cIsomerization experiments;dReaction of alkyne with oxalate;eStoichiometric reaction of isolated Ni(II) complex.dtbbpy= 4,4′-di-tert-butyl-2,2′-dipyridyl 12 and Supplementary Table 4 ). Therefore, we expected that a catalytic Ni 0/I/III pathway, proceeding via capture of alkenyl radical by Ni(0), followed by oxidative addition and then reductive elimination, could be operative in this metallaphotoredox manifold (Fig. 2 ). Fig. 5 Mechanistic studies. a Time course studies; b UV–Vis absorption spectrometry; c Isomerization experiments; d Reaction of alkyne with oxalate; e Stoichiometric reaction of isolated Ni(II) complex. dtbbpy = 4,4′-di- tert -butyl-2,2′-dipyridyl Full size image In conclusion, we have developed a generic protocol for the intermolecular, regioselective, syn -alkylarylation of terminal alkynes with tertiary alkyl oxalates through a synergistic merger of photoredox and nickel catalysis. A one-pot, three-step sequence, involving radical addition, transition-metal-based coupling, and alkene isomerization, proceeds with high efficiency under the light-induced mild conditions. This manifold forges two vicinal C–C bonds, yielding a variety of trisubstituted alkenes with excellent regioselectivity and syn -stereoselectivity. We expect that the operational simplicity and generality of this methodology and readily availability of the starting materials will allow it to enjoy extensive application in the area of organic chemistry. General procedure for the syn -selective alkylarylataion reaction To a flame dried 8 mL reaction vial was charged with Ir[dF(CF 3 )ppy] 2 (dtbbpy)(PF 6 ) (0.003 mmol, 3 mol%), NiCl 2 •DME (0.02 mmol, 20 mol%), 4,4′-di- tert -butyl-2,2′-dipyridyl (0.02 mmol, 20 mol%), aryl bromide (0.2 mmol, 2.0 equiv. ), and cesium alkyl oxalate (0.15 mmol, 1.5 equiv.). The vial was capped. After evacuated and backfilled nitrogen three times, DMSO [0.05 M] was added via a syringe, followed by the addition of terminal alkyne (0.1 mmol, 1.0 equiv.). The reaction mixture was irritated with a 90 W blue LED, with cooling from a fan (36 °C). After 18 h, the reaction was quenched with H 2 O, extracted with ethyl acetate. The combined organic layers were dried with MgSO 4 , filtered, and concentrated in vacuo. The crude material was purified by flash chromatography to afford the products. See Supplementary Methods for further experimental details.